Temporal niche promotes biodiversity during adaptive radiation Understanding mechanisms underlying the origin and maintenance of biodiversity is a central goal of modern ecological and evolutionary research. Ecologists have recognized the potentially important role of temporal niche in promoting species coexistence and diversity, yet little is known about how temporal niche affects the evolution of biodiversity. Here we show that temporal niche strongly influences biodiversity dynamics in rapidly evolving bacteria. An ancestral bacterium quickly diversifies when provided with constant spatial niche opportunities or when experiencing temporal niche dynamics. However, only in communities with temporal niches, which promote frequency-dependent selection and the positive growth of new mutants, is the accumulated phenotypic diversity able to persist. Overall, the presence of temporal niche opportunities eliminates the overshooting dynamics of adaptive radiation typically seen in this and other systems. These results suggest that temporal niche may have an essential role in the maintenance of biodiversity over evolutionary time. For decades, biologists have sought to understand mechanisms underlying high biodiversity observed in many of the Earth’s ecosystems [1] , [2] , [3] . The theory of temporal niche dynamics (TND) suggests that temporal variation in niche availability allows the storage effect to operate, buffering species against extinction [4] , [5] . Increased species coexistence in fluctuating environments has been documented for both natural [6] , [7] , [8] and experimental [9] , [10] communities, and has, in a few cases, been explicitly linked to TND [6] , [11] . In parallel, diversification under fluctuating selection has been of much interest for evolutionary biologists [12] , [13] , [14] . However, while TND has received some theoretical attention in this context [15] , [16] , little empirical knowledge exists on how it affects biodiversity dynamics in systems where ongoing evolution contributes to biodiversity [17] . We hypothesize that because TND modulates ecological interactions that often provide the selective force for evolution, it may affect the emergence and maintenance of biodiversity over evolutionary timescales. Testing this idea is difficult in many systems, given the generally long period of biodiversity evolution and inadequate knowledge on the niches of evolved lineages. Such tests, however, are feasible using microbial lineages undergoing rapid adaptive radiation, which can give rise to new phenotypes/species adapted to different niches in a short period of time. We investigated biodiversity dynamics in the rapidly diversifying Pseudomonas fluorescens SBW25 populations [18] , [19] . Previous research has shown that a suite of environmental factors, such as disturbance [20] , [21] and productivity [19] , affect the diversification of this bacterium. A key advantage of this experimental system is that rapid adaptive radiation produces ecotypes with different niche preferences [18] , [19] , which allowed us to directly manipulate the temporal availability of these niches and link coexistence with TND, an approach that has not been taken previously. When introduced into static microcosms, the ancestral P. fluorescens ecotype—smooth morph (SM) that occupies the broth phase—diversifies and generates two niche-specialists: the wrinkled spreader (WS) ecotype that colonizes the air-broth interface, and the fuzzy spreader (FS) ecotype that inhabits the bottom of microcosms. Competition for oxygen, whose concentration decreases towards the bottom of static microcosms, is thought to be an important factor in driving this niche differentiation [18] . Additional variations also exist within each ecotype. Within WS, for example, small-WS, large-WS, wheel-WS and SM-like-WS subtypes may also emerge [22] , driven likely by adaptation to micro-niches [23] . These P. fluorescens phenotypes are genetically determined and can be readily distinguished on agar plates [18] , [22] . Each phenotype may be considered as analogous to a biological species as P. fluorescens reproduces asexually with a low recombination rate [18] , [22] . The spatially structured niches provided by the static incubation are favourable for WS and FS, and crucial for SM diversification. Shaking of microcosms eliminates spatial niches (for example, the oxygen gradient), making it difficult for SM to diversify. Therefore, temporal shifting between static and shaking conditions provides temporal niche opportunities for P. fluorescens communities [18] . Here we examine biodiversity dynamics in a laboratory experiment in which evolving P. fluorescens populations were incubated with or without temporal niche (see Methods). We show that the availability of temporal niche is critical for the maintenance of the evolved P. fluorescens phenotypic diversity, via the mechanism of promoting negative frequency-dependent selection. These results suggest that TND have the potential to strongly influence biodiversity dynamics over evolutionary time. Temporal niches and phenotypic diversity As in previous studies [22] , [23] , new phenotypes, including small-WS, large-WS, wheel-WS, SM-like-WS and FS, quickly emerged in static microcosms (all phenotypes detected by day 4; Figs 1a and 2a ). This rapid increase in phenotypic richness, however, was followed by a slower decline, as some of the emerged phenotypes were later competitively excluded [23] ( Fig. 1a ). Such overshooting dynamics are predicted by theory [24] , and have been previously reported for this experimental system [22] , [23] , as well as adaptive radiations in nature [6] , [25] , [26] . By contrast, diversification in microcosms experiencing constant shaking was much slower, presumably due to the lack of spatial niches for new phenotypes [18] , resulting in the slow accumulation of phenotypes over the duration of the experiment ( Figs 1a and 2b ). The presence of TND, however, led to different biodiversity dynamics. Although rapid diversification also occurred in TND microcosms, most of the derived phenotypes, including FS and multiple WS phenotypes, persisted afterwards in these microcosms ( Fig. 2c ). Rather than exhibiting overshooting dynamics, phenotypic richness here approached an asymptote, albeit in an oscillatory fashion, during the second half of the experiment ( Fig. 1a ). As a result, final phenotypic richness was significantly greater with than without temporal niche structure ( Fig. 1a ). The two TND treatments (shaking-static and static-shaking) did not differ in final phenotypic richness. 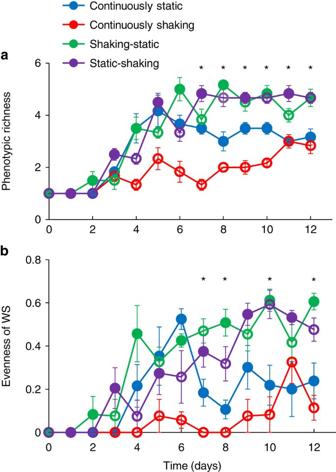Figure 1: Biodiversity dynamics in the temporal niche experiment. (a) Phenotypic richness ofP. fluorescens; (b) evenness of WS phenotypes. Solid and open circles indicate that microcosms were incubated under the static and shaking condition on the day before sampling, respectively. Values are mean±s.e.m. (n=6). Asterisks indicate that the values in at least one of the two TND treatments (shaking-static and static-shaking) are significantly greater than the values in the continuously static treatment in a Tukey’s Honestly Significant Difference test (P<0.05). The effect sizes (η2) of analysis of variance of phenotypic richness and WS evenness on day 12 are 0.62 and 0.53, respectively. Figure 1: Biodiversity dynamics in the temporal niche experiment. ( a ) Phenotypic richness of P. fluorescens ; ( b ) evenness of WS phenotypes. Solid and open circles indicate that microcosms were incubated under the static and shaking condition on the day before sampling, respectively. Values are mean±s.e.m. ( n =6). Asterisks indicate that the values in at least one of the two TND treatments (shaking-static and static-shaking) are significantly greater than the values in the continuously static treatment in a Tukey’s Honestly Significant Difference test ( P <0.05). The effect sizes ( η 2 ) of analysis of variance of phenotypic richness and WS evenness on day 12 are 0.62 and 0.53, respectively. 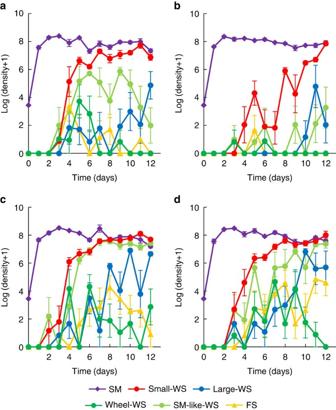Figure 2: Population dynamics of each phenotype in the four experimental treatments. (a) Continuously static; (b) continuously shaking; (c) shaking-static; (d) static-shaking. Population density data (CFU ml−1) were log10(x+1)-transformed. Values are mean±s.e.m. (n=6). Full size image Figure 2: Population dynamics of each phenotype in the four experimental treatments. ( a ) Continuously static; ( b ) continuously shaking; ( c ) shaking-static; ( d ) static-shaking. Population density data (CFU ml −1 ) were log 10 ( x +1)-transformed. Values are mean±s.e.m. ( n =6). Full size image We further examined diversity patterns within the group of WS phenotypes, which made up the majority of phenotypic diversity in the population ( Fig. 2 ). The dynamics of WS phenotype evenness, calculated as Pielou’s J ' [27] , largely mirrored those of overall phenotypic richness ( Fig. 1b ). WS evenness in static microcosms exhibited overshooting dynamics, with the later decline in evenness associated with the extinction or reduced abundance of several WS phenotypes. This can be explained by within-niche competition, where small-WS attained numerical dominance within this group of niche specialists [23] ( Fig. 2a ). In contrast, in TND microcosms, as several WS phenotypes attained appreciable abundance while coexisting with small-WS, overshooting in evenness was not observed ( Fig. 2c ). WS fitness and frequency-dependent selection Our experimental results indicate that TND promoted biodiversity mainly by allowing more phenotypes sharing similar niches (that is, WS phenotypes) to coexist. Both static and shaking conditions appeared to be important: while the availability of spatial niches under static incubation allowed the emergence of different WS phenotypes, shaking apparently prevented the loss of some of the WS phenotypes that otherwise would be driven to extinction by small-WS. This increased coexistence under TND may be caused by frequency-dependent selection [4] , [5] , which is known to operate among some P. fluorescens phenotypes [18] , [28] , [29] . To explore the possibility that frequency-dependent selection operates among WS subtypes, we conducted a second experiment with four wild-type WS phenotypes and one lacZ-marked SM phenotype, allowing each wild-type WS phenotype to be initially more abundant than others (see Methods). The lacZ-marked SM gives rise to WS mutants whose colonies exhibit a distinct blue colour on agar plates with X-gal, which can be used to distinguish them from wild-type WS colonies [22] . We estimated the fitness of the initially dominant WS phenotypes relative to other WS phenotypes after 2-day incubations under either shaking or static conditions (according to Equation 1 in the Methods). We found that while the initially dominant WS phenotypes attained greater dominance in static microcosms, their fitness was significantly reduced in shaken microcosms, such that the relative fitness for none of the four phenotypes was positive ( Figs 3a and 4 ). In addition, only in shaken microcosms was the fitness of the initially dominant WS phenotypes negatively correlated with their initial frequency ( Fig. 3b ). These signatures of frequency-dependent selection suggest that shaking provided fitness advantage for rare WS phenotypes relative to common ones. Note that the absolute fitness of each WS phenotype was still smaller under shaking relative to static conditions, presumably because shaking eliminated their preferred niche. Moreover, only under shaken incubation was in situ mutation from lacZ-marked SM phenotype to WS detected ( Fig. 5 ), indicating that shaking favored new WS mutants. Together, these results suggest that shaking, while eliminating the niche of WS phenotypes, promoted their coexistence in the TND microcosms. 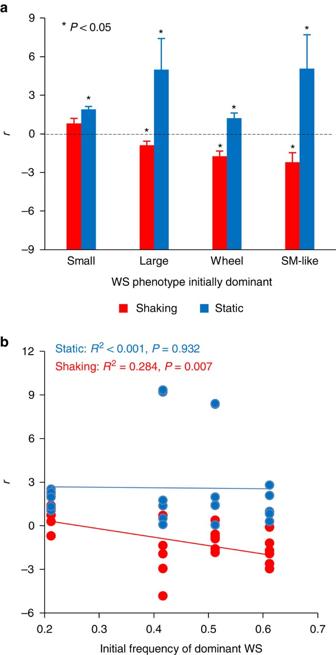Figure 3: Fitness of the dominant WS phenotype in the shaken and static microcosms. Fitness is calculated as the difference in the Malthusian parameter (r) between the initially dominant and other WS phenotypes according to Equation 1. (a) Fitness of each phenotype in the shaking and static microcosms. Values are mean+s.e.m. (n=6). Asterisks indicate treatments where the values are different from zero according to one samplet-test (P<0.05). Note that the fitness of small-WS under shaking was not significantly different from zero, whereas fitness in other treatments all differed from zero. (b) The relationship between the frequency of initially dominant WS phenotype and its fitness under shaking and static conditions. The linear regressions are shown with data. Figure 3: Fitness of the dominant WS phenotype in the shaken and static microcosms. Fitness is calculated as the difference in the Malthusian parameter ( r ) between the initially dominant and other WS phenotypes according to Equation 1. ( a ) Fitness of each phenotype in the shaking and static microcosms. Values are mean+s.e.m. ( n =6). Asterisks indicate treatments where the values are different from zero according to one sample t -test ( P <0.05). Note that the fitness of small-WS under shaking was not significantly different from zero, whereas fitness in other treatments all differed from zero. ( b ) The relationship between the frequency of initially dominant WS phenotype and its fitness under shaking and static conditions. The linear regressions are shown with data. 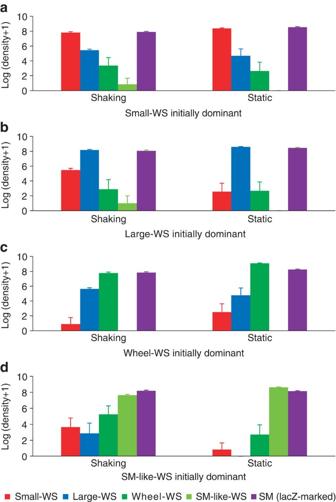Figure 4: Population density of each phenotype in the WS fitness experiment. (a) small-WS initially dominant; (b) large-WS initially dominant; (c) wheel-WS initially dominant; (d) SM-like-WS initially dominant. Population density data (CFU ml−1) were log10(x+1)-transformed. Values are mean+s.e.m. (n=6). Full size image Figure 4: Population density of each phenotype in the WS fitness experiment. ( a ) small-WS initially dominant; ( b ) large-WS initially dominant; ( c ) wheel-WS initially dominant; ( d ) SM-like-WS initially dominant. Population density data (CFU ml −1 ) were log 10 ( x +1)-transformed. Values are mean+s.e.m. ( n =6). 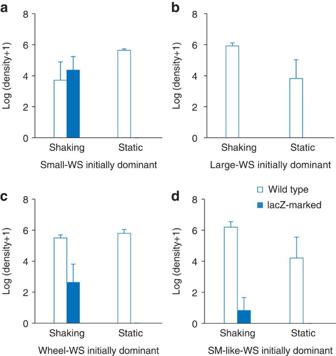Figure 5: The density of nondominant WS phenotypes of wild and lacZ-marked types in the shaken and static microcosms. (a) Small-WS initially dominant; (b) large-WS initially dominant; (c) wheel-WS initially dominant; (d) SM-like-WS initially dominant. Data (CFU ml−1) were log10(x+1)-transformed. Values are mean+s.e.m. (n=6). Full size image Figure 5: The density of nondominant WS phenotypes of wild and lacZ-marked types in the shaken and static microcosms. ( a ) Small-WS initially dominant; ( b ) large-WS initially dominant; ( c ) wheel-WS initially dominant; ( d ) SM-like-WS initially dominant. Data (CFU ml −1 ) were log 10 ( x +1)-transformed. Values are mean+s.e.m. ( n =6). Full size image Using a model organism undergoing rapid adaptive radiation, we examined the hypothesis that TND affects the evolution of biodiversity. Although we did not find evidence of TND altering the emergence of diversity, our experiments clearly show that it functioned to maintain evolved diversity and stabilize its dynamics. To our knowledge, this is the first experimental demonstration of TND promoting biodiversity over evolutionary time. One notable characteristic of TND in our experiment is that static conditions facilitated the generation of diversity by offering spatial niches, whereas shaking prevented the loss of evolved diversity by promoting negative frequency-dependent selection between the WS phenotypes. Previous studies have revealed that negative frequency-dependent selection also operated between SM and WS phenotypes under static conditions, facilitating their coexistence [18] , [23] , [28] . This scenario differs from the more commonly considered situations where the TND effect operates as the result of different species being favored by different niches associated with different environmental conditions. Nevertheless, both static and shaking conditions were essential for the persistence of evolving diversity, in a similar manner as alternations in environmental conditions that favour different species were essential for species coexistence over ecological time. The negative frequency-dependent selection among the WS phenotypes under shaken conditions warrants some explanation. Frequency-dependent selection arose probably because subordinate WS genotypes faced strong competition in their niche (air-broth interface) housing concentrated small-WS populations under static conditions, but experienced weakened competition from diffused small-WS populations under shaking conditions. In addition, for essentially the same reason, shaking may have facilitated the coexistence of WS phenotypes via increasing the fitness of newly evolved nondominant WS individuals. In the context of the storage effect [4] , the first scenario would generate covariance between competition and environment, and the second scenario would contribute to buffered population growth (that is, the supply of new mutants buffering populations against extinction) in addition to that afforded by overlapping generations [16] , [30] . Several features of our experimental regime are worth noting. First, alternation between static and shaking conditions in our experiment not only created temporal niche opportunities, but also altered the average environmental conditions. As it is impossible to create a constant environment equivalent to the average of static and shaking conditions, the possibility that increased diversity may be partly driven by changes in average conditions cannot be completely excluded. The demonstrated role of static conditions for diversity generation and of shaking conditions for diversity maintenance, however, point to the importance of TND. Second, our TND microcosms were shifted between static and shaking conditions every 24 h, which allowed frequency-dependent selection to exert its force under shaking conditions while mitigating competitive exclusion of nondominant WS populations under static conditions. In a related experiment, Massin and Gonzalez [21] studied the effects of short-term (2 min duration) pulse disturbance, in the form of shaking the otherwise static microcosms, on P. fluorescens diversification. Contrasting with our results, their experiment showed that periodic disturbance slowed diversification, presumably because the short-term shaking eliminated spatial niches without incurring frequency dependence. Third, daily dilution was used to propagate P. fluorescens populations in our experiment. Buckling et al. [20] reported that the frequency of dilution affected P. fluorescens phenotypic diversity, such that diversity exhibited a unimodal relationship with dilution frequency in static microcosms. Obviously, experiments with different dilution frequencies are needed to further test the robustness of our results. Note that daily dilution in our experiment (see Methods) may have also resulted in different diversity dynamics than previously reported for P. fluorescens batch cultures [18] . Our results demonstrate that TND can strongly influence evolutionary dynamics of biodiversity. Given the prevalence of environmental fluctuations that offer temporal niche opportunities at various timescales in nature [31] , [32] , this result has important implications for understanding diversification patterns in many natural systems. For example, whereas overshooting dynamics are frequently encountered when studying adaptive radiation in nature [25] , [26] , many lineages have diversified without showing an apparent decline in diversity [32] , [33] . Although alternative hypotheses exist [22] , [31] , our results suggest that TND may potentially explain the maintenance of the accumulated biodiversity over evolutionary time. Bacterial cultivation We cultivated P. fluorescens SBW25 (wild-type and lacZ-marked) in 25 ml loosely capped test tubes containing 6 ml King’s Medium B (KB) on a shaker (250 r.p.m.) at 28 °C. After 48 h, we plated the cultures on KB agar plates and incubated the plates at 28 °C for another 48 h. One wild-type SM colony was isolated for use in the experiments; one lacZ-marked SM colony was isolated and cultivated in KB overnight and stored in 15% glycerol at −80 °C. Before setting up the SM stock culture, we thawed the P. fluorescens culture previously frozen at −80 °C, and plated it on agar. We then isolated one 2-day-old SM colony on the agar plate, and introduced it into a test tube with 6 ml KB. After incubating the culture for 2 h, we introduced 10 μl of this culture into each experimental microcosm. Experimental protocols Microcosms were 25 ml capped test tubes containing 6 ml KB. The initial SM density in each microcosm was ~10 3 colony-forming units (CFU) per ml. Microcosms without temporal niche were incubated under continuously static or shaking conditions. Microcosms with temporal niche were alternated between shaking and static conditions every 24 h, a period that permits P. fluorescens phenotypes to grow and interact for multiple (10–12) generations. Two different regimes of temporal niche were used: one under shaking incubation on odd days and static incubation on even days (shaking-static), and the other with the reverse sequence (static-shaking). The two regimes allowed us to discern if initial environmental conditions (static or shaking) matter for biodiversity evolution. We propagated P. fluorescens populations by transferring 1% of the content of each microcosm into a fresh microcosm daily, and quantified the abundance of each phenotype afterwards. Under the static condition, microcosms were kept at 28 °C without shaking; under the shaking condition, microcosms were placed on a shaker (250 r.p.m.) at 28 °C. Each treatment was replicated six times. The experiment ended after 12 days. Quantifying phenotypic density and diversity The density of each phenotype was measured after the daily transfer. The sample from each microcosm was spread onto KB agar plates after serial dilutions. A total of six P. fluorescens phenotypes, SM, FS, small-WS, large-WS, wheel-WS and SM-like-WS, were identified and the number of colonies of each phenotype was recorded. Phenotypic richness was the number of phenotypes detected in the sample, and the evenness of WS phenotypes was calculated as Pielou’s J ' [27] . We assessed the treatment effects on phenotypic richness and WS evenness using analysis of variance, followed by Tukey’s Honestly Significant Difference tests. WS fitness experiment From the temporal niche experiment, we isolated four WS phenotypes derived from the wild-type SM and preserved them in 15% glycerol at −80 °C. Before the experiment, we established separate stock cultures for the four WS phenotypes and lacZ-marked SM in microcosms with 6 ml KB and incubated them overnight. We initiated the experiment with highly uneven WS phenotype densities such that the ratio of the dominant WS, three nondominant WS and lacZ-marked SM was 1,000:1:1:1:1,000 (initial density: 10 6 :10 3 :10 3 :10 3 :10 6 CFU ml −1 ). The experiment had four treatments each with a different WS phenotype being initially dominant. Each treatment was replicated six times. Microcosms were under either static or shaking incubation for 2 days at 28 °C. Thereafter, we sampled each microcosm to quantify the final abundance of each phenotype. We calculated the relative fitness of the initially dominant WS using the ratio of Malthusian parameter ( r ), according to equation 1. We conducted a two-tailed t -test to compare the difference in r between shaking and static incubations for each of the four experimental treatments. How to cite this article: Tan, J. et al. Temporal niche promotes biodiversity during adaptive radiation. Nat. Commun. 4:2102 doi: 10.1038/ncomms3102 (2013).